Lithium carbonate-promoted mixed rare earth oxides as a generalized strategy for oxidative coupling of methane with exceptional yields 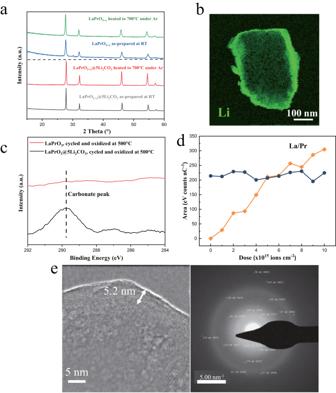Fig. 1: Ex-situ and in-situ spectroscopic characterizations for LaPrO3+x@5Li2CO3. aIn-situ XRD on LaPrO3+x@5Li2CO3under air at 700 °C;bEx-situ TEM-EELS on LaPrO3+x@5Li2CO3in vacuum;cIn-situ XPS on LaPrO3+xand LaPrO3+x@5Li2CO3, both LaPrO3+xand LaPrO3+x@5Li2CO3were reduced with diluted methane at 700 °C and re-oxidized with diluted oxygen at 500 °C in the in-situ XPS chamber;dQuasi in-situ HS-LEIS on LaPrO3+x@5Li2CO3treated in 600 °C under 10% O2in a pretreatment chamber;eIn-situ TEM and electron diffraction of LaPrO3+x@5Li2CO3at 700 °C under diluted O2. The oxidative coupling of methane to higher hydrocarbons offers a promising autothermal approach for direct methane conversion, but its progress has been hindered by yield limitations, high temperature requirements, and performance penalties at practical methane partial pressures (~1 atm). In this study, we report a class of Li 2 CO 3 -coated mixed rare earth oxides as highly effective redox catalysts for oxidative coupling of methane under a chemical looping scheme. This catalyst achieves a single-pass C 2+ yield up to 30.6%, demonstrating stable performance at 700 °C and methane partial pressures up to 1.4 atm. In-situ characterizations and quantum chemistry calculations provide insights into the distinct roles of the mixed oxide core and Li 2 CO 3 shell, as well as the interplay between the Pr oxidation state and active peroxide formation upon Li 2 CO 3 coating. Furthermore, we establish a generalized correlation between Pr 4+ content in the mixed lanthanide oxide and hydrocarbons yield, offering a valuable optimization strategy for this class of oxidative coupling of methane redox catalysts. Efficient, single-step conversion of methane into value-added chemicals has been a critical challenge in C1 chemistry. Among the various conversion methods, oxidative coupling of methane (OCM), which employs gas-phase molecular O 2 to generate higher hydrocarbons (C 2+ ) in an autothermal process, has garnered significant research attention since its inception in the 1980s [1] . Over the past 40 years, ~2000 OCM catalysts have been identified for OCM through experimental screening and/or with the assistance of machine learning [1] , [2] , [3] , [4] . Among the investigated materials, top-performing candidates predominantly fall within two distinct catalyst families: the unsupported Li-MgO mixed oxide and the supported Mn-Na 2 WO 4 /SiO 2 . The Li-MgO bulk mixed oxide catalyst was first reported by Lunsford et al. in 1985 and achieved up to 19% C 2+ yield at 720 °C [5] , [6] . While various optimizations have been conducted on this catalyst, the C 2+ yield has yet to exceed 20% [7] , [8] . Moreover, catalyst deactivation issues persist due to evaporation of lithium in the form of LiOH [9] , [10] . In 1992, Fang et al. reported that the supported Mn-Na 2 WO 4 /SiO 2 catalyst demonstrated 23.9% C 2+ yield at 800 °C [11] . Extensive studies were performed on this catalyst including material screening [12] , surface and bulk structural characterization [13] , reaction pathway and mechanism modeling [14] , and reactor optimization [15] . While deeper mechanistic insights into these catalyst families have been obtained in recent years [14] , [16] , [17] , the observed C 2+ yield has not exceeded 30% for the Mn-Na 2 WO 4 /SiO 2 catalyst family, which showed satisfactory stability in general. Outside of the Li-MgO and Mn-Na 2 WO 4 /SiO 2 catalyst families, La 2 O 3 -CeO 2 nanofibers have exhibited a C 2+ yield of ~20% at the relatively low temperature of 520 °C [18] . By maximizing all the desired reaction rates and optimizing thermochemistry for all the surface species on an idealized catalyst, Green et al. predicted, through kinetic modeling, that the C 2+ yield would limit to ~28% in catalytic OCM with O 2 -cofeed [19] . This is consistent with the experimentally reported yields to date. To address the yield limitations from co-feeding methane and gaseous O 2 , research has also been conducted on spatially and/or temporally separating the contact of methane and O 2 for OCM. Up to 34.7% C 2+ yield was reported at 900 °C in diluted methane ( P CH4 < 0.5 atm) using a catalytic membrane reactor composed of a mixed-conductive Ba 0.5 Ce 0.4 Gd 0.1 Co 0.8 Fe 0.2 O 3−δ membrane and a supported Mn-Na 2 WO 4 /SiO 2 catalyst. However, rapid membrane degradation was observed, a common challenge for membrane-based OCM at such elevated temperatures [20] . Lattice oxygen-based OCM has also been performed under a chemical-looping (CL) mode, which utilizes a reducible metal oxide operated through cyclic redox steps under alternating methane and O 2 environments [21] , [22] . Gaffney et al. pioneered the concept of chemical looping-OCM (CL-OCM) and reported that a Na impregnated Pr 6 O 11 catalyst achieved up to 16% C 2+ yield at 775 °C [23] . The chemical looping mode utilizes the redox between Pr 4+ and Pr 3+ and demonstrated ~4% higher C 2+ yield than the O 2 -cofeed mode. More recently, Fan et al. proposed the idea of CL-OCM by designing a Li and W co-doped Mg 6 MnO 8 redox catalyst that exhibited 28.6% C 2+ yield at 850 °C [24] , [25] . To date, more than 10,000 articles have been published on OCM. However, none of the prior studies have demonstrated >30% C 2+ yield with satisfactory stability. Moreover, most of these studies were carried out with highly diluted methane, which would not be suitable for practical applications. Based on experimental data coupled with kinetic analyses, Labinger et al. argued that higher methane partial pressures would lead to severe yield penalties [26] . On the other hand, it has been estimated that for OCM to achieve commercial viability, a C 2+ yield exceeding 30–35% at practical partial pressures (~1 atm) is required [27] . As such, a gap clearly exists between reported academic research results and industrial application [28] . From a mechanistic aspect, various active sites or active species have been postulated to be responsible for methane activation. Taking Li-MgO as a model catalyst, early studies by Lunsford et al. suggested that Li + O − is the active site based on electron spin resonance (EPR) of quenched catalysts in the presence of O 2 with the g ⊥ = 2.054 signal [5] , [29] . Based on the O 1 s shoulder observed at 533 eV in ex-situ X-ray photoelectron spectroscopy (XPS) using a spectrometer equipped with a pretreatment chamber, Stair et al. argued for the presence of peroxide or Li + O − species in the surface region (<3 nm) [30] . The presence of peroxides for OCM on a related, unsupported Ba/MgO mixed oxide catalyst was reported by Lunsford et al. on the basis of in-situ Raman (with the BaO 2 band at 842 cm −1 ) and ex-situ XPS (with the O 1 s peak at 531 eV) [31] , [32] . While the presence of peroxides was largely confirmed, the necessity for Li + O − sites was questioned by subsequent studies involving both experimental work and quantum chemistry calculations [33] , [34] . These studies argued that Mg 2+ O 2− sites or defective MgO surfaces are responsible for methane activation, and Li only acts as a structural modifier instead of an active center [33] , [34] . The search for active sites in the supported Mn-Na 2 WO 4 /SiO 2 was similarly challenging. A number of earlier studies, mostly through ex-situ measurements, proposed that the active sites are either Na-O-Mn, Na-O-W or other bonds belonging to bulk crystalline phases selected from the Mn-Na-W-O components [35] . More recently, Wachs et al. conducted in-situ Raman studies and demonstrated that none of the abovementioned crystalline phases are actually present at the OCM reaction temperature (900 °C), and the active site for methane activation are isolated, pseudotetrahedral Na-coordinated WO 4 surface sites (Na-WO 4 ) on the SiO 2 support [13] , [14] , [16] . Through separate studies, Takanabe and Tao et al. detected the presence of peroxide species for both supported K 2 WO 4 /SiO 2 and Na 2 WO 4 /SiO 2 [36] , [37] catalysts with in-situ XPS. Using laser induced fluorescence (LIF) measurements. Tao further proposed that the presence of near-surface peroxides can lead to the formation of hydroxyl radicals for methane activation. Given the potential role of surface/subsurface peroxide species and the redox properties of praseodymium oxides in the context of chemical looping [23] , the current study focuses on Pr-containing lanthanide oxides with a Li 2 CO 3 promoter for CL-OCM. Li 2 CO 3 was selected because it has good \({{{{{{\rm{O}}}}}}}_{2}^{2-}\) solubility and conductivity, and was previously reported to be effective for ethane activation [38] . Unsupported bulk mixed oxides containing Pr and another lanthanide cation, on the other hand, can beneficially modify the redox properties of Pr 4+ /Pr 3+ [23] . In the present study, a series of Pr-containing lanthanide oxides with a thin surface film of Li 2 CO 3 (LnPrO 3+x @Li 2 CO 3 , Ln = La, Eu, Ho, Dy, Sm, and Nd) for CL-OCM were synthesized and characterized. 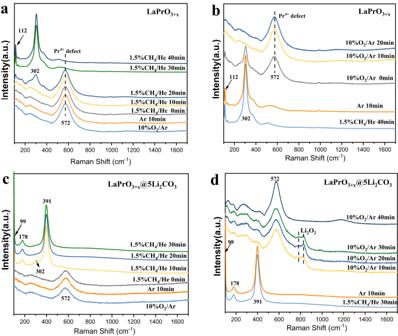Fig. 2: In-situ Raman for LaPrO3+xand LaPrO3+x@5Li2CO3. In-situ Raman foraLaPrO3+xreduction at 700 °C,bLaPrO3+xreoxidation at 700 °C,cLaPrO3+x@5Li2CO3reduction at 700 °C,dLaPrO3+x@5Li2CO3reoxidation at 700 °C. This family of materials exhibited up to 30.6% single-pass C 2+ yield with stable performance at 700 °C. The roles of the mixed oxide core and Li 2 CO 3 shell, as well as the interplays among the Pr oxidation state, active peroxide formation upon Li 2 CO 3 coating, and OCM performance were determined by ex-situ X-ray absorption near edge structure (XANES), in-situ Raman, in-situ X-ray diffraction (XRD), in-situ XPS, and quantum chemistry calculations. Structures of catalyst bulk phase and surface region under different environments While all the Li 2 CO 3 promoted LnPrO 3+x oxides (Ln = La, Eu, Ho, Dy, Sm, Nd) were active for OCM (as will be discussed in later sections), LaPrO 3+x @5Li 2 CO 3 (5 refers to 5 wt.% Li 2 CO 3 loading) was selected as a representative redox catalyst for detailed characterizations since it showed excellent performance and La is a relatively abundant rare earth element. The LaPrO 3+x @5Li 2 CO 3 redox catalyst consists of a core-shell structure. The core consists of the crystalline LaPrO 3+x bulk phase as shown by in-situ XRD at 700 °C (Fig. 1a ). The crystalline LaPrO 3+x core is covered by a thin Li 2 CO 3 shell as revealed by (i) spatial distribution of Li in the mapping of the ex-situ TEM-EELS analysis on a catalyst particle (Fig. 1b ), (ii) surface enrichment of carbon with TEM-EDS (Supplementary Fig. S1 ) whereas carbonate-free LaPrO 3+x does not exhibit a XPS signal for carbon (Fig. 1c ), (iii) presence of carbon and lithium in the surface region of LaPrO 3+x @5Li 2 CO 3 with in-situ XPS (Supplementary Fig. S2 ), and (iv) absence of Pr and La on the outermost surface layer (0.3 nm) as revealed by high sensitivity - low energy ion scattering (HS-LEIS) analysis of the surface, and the increase in the La and Pr signals with sputtering depth (Fig. 1d ). The thin Li 2 CO 3 shell (<5 nm) is amorphous and lacks long range order. Therefore, its signal does not appear in the in-situ XRD pattern (Fig. 1a ). Furthermore, bulk Li 2 CO 3 melts at 723 °C, suggesting that the surface layer is likely be in a molten state under the OCM reaction conditions (~700 °C) given the lower melting temperatures of thin films [38] . The in-situ TEM analysis (Fig. 1e ) further verifies the morphology and composition of the LaPrO 3+x @5Li 2 CO 3 catalyst, which consists of a crystalline LaPrO 3+x core enveloped by a thin amorphous Li 2 CO 3 shell at 700 °C. Fig. 1: Ex-situ and in-situ spectroscopic characterizations for LaPrO 3+x @5Li 2 CO 3 . a In-situ XRD on LaPrO 3+x @5Li 2 CO 3 under air at 700 °C; b Ex-situ TEM-EELS on LaPrO 3+x @5Li 2 CO 3 in vacuum; c In-situ XPS on LaPrO 3+x and LaPrO 3+x @5Li 2 CO 3 , both LaPrO 3+x and LaPrO 3+x @5Li 2 CO 3 were reduced with diluted methane at 700 °C and re-oxidized with diluted oxygen at 500 °C in the in-situ XPS chamber; d Quasi in-situ HS-LEIS on LaPrO 3+x @5Li 2 CO 3 treated in 600 °C under 10% O 2 in a pretreatment chamber; e In-situ TEM and electron diffraction of LaPrO 3+x @5Li 2 CO 3 at 700 °C under diluted O 2 . Full size image The relationship between near-surface peroxide and Pr 4+ Given that CL-OCM reactions proceed through cyclic removal (OCM step) and replenishment (re-oxidation step) of lattice oxygen from bulk reducible oxides in the redox catalyst, the dynamics of the bulk LaPrO 3+x phase for LaPrO 3+x and LaPrO 3+x @5Li 2 CO 3 under oxidizing and methane reducing conditions were further monitored with in-situ XRD, Raman and XPS at 700 °C. The oxidized Li-free bulk LaPrO 3+x mixed oxide is present as cubic-LaPrO 3.33 and transforms to a mixture of cubic-La 2 O 3 and cubic-Pr 2 O 3 after methane reduction (see in-situ XRD in Supplementary Fig. S3 ). This is corroborated by the corresponding in-situ Raman spectra (Fig. 2 a, b), showing that the oxidized cubic-LaPrO 3.33 phase (572 cm −1 ) is reduced to cubic-La 2 O 3 and cubic Pr 2 O 3 (112 and 302 cm −1 ). Westermann et al. assigned the band at 572 cm −1 to Pr 4+ defects [39] . Re-oxidation converts the reduced phase back to the initial oxidized state. Cubic-LaPrO 3+x is also present in the oxidized LaPrO 3+x @5Li 2 CO 3 catalyst, but it reversibly transforms to the bulk hexagonal-LaPrO 3+x phase after methane reduction. This is confirmed by in-situ XRD in Supplementary Fig. S3 and in-situ Raman spectra in Fig. 2c, d, where the oxidized bulk c-LaPrO 3+x (572 cm −1 ) was reduced to the bulk h-LaPrO 3+x (178 and 392 cm −1 ). Thus, the amorphous Li 2 CO 3 shell affects the structure of the bulk LaPrO 3+x phase under the OCM conditions. The presence of the Li 2 CO 3 shell also resulted in the formation of peroxide species (O 2 2− : in-situ Raman band at ~850 cm −1 characteristic of Li 2 O 2 ) [40] during the transient oxidation of the reduced LaPrO 3+x @5Li 2 CO 3 mixed oxide. The absence of peroxide species for the Li-free LaPrO 3+x and the presence of the peroxide species for LaPrO 3+x @5Li 2 CO 3 suggest that the peroxide species are associated with the thin Li 2 CO 3 shell. It is noted that the surface area of Li 2 CO 3 promoted LaPrO 3+x is quite low (~1 m 2 /g, Supplementary Table S1 summarizes the surface areas of bare LaPrO 3+x and LaPrO 3+x with different Li 2 CO 3 loadings), the ability for Raman to detect the peroxide species in this low surface area assay suggests that the detected peroxide signal cannot just be surface bound. Rather, contributions from bulk peroxide species, e.g. peroxides dissolved/incorporated in the amorphous Li 2 CO 3 shell, is more likely. We also note that Raman did not detect Li 2 CO 3 peaks from this sample, this is probably due to its low loading (5 wt.%) and the peak broadening effect of amorphous carbonate as the temperature increases [41] . This peak broadening effect was confirmed via an in-situ Raman experiment on LaPrO 3+x @5Li 2 CO 3 under 5%CO 2 (balance Ar) with temperature ramping up from 120 to 700 °C. As shown in Supplementary Fig. S4a , LaPrO 3+x @5Li 2 CO 3 exhibited a clear surface carbonate peak between 1100–1300 cm −1 . This peak, however, tends to be broadened and smoothed out when the temperature gradually ramped up to 700 °C. We note that this broadening effect is not likely due to the thermal decomposition of Li 2 CO 3 since the presence of 5 vol.% CO 2 would inhibit carbonate decomposition from a thermodynamic standpoint. We have also compared ex-situ Raman under air in room temperature for LaPrO 3+x @3Li 2 CO 3 , LaPrO 3+x @5Li 2 CO 3 and LaPrO 3+x @10Li 2 CO 3 . All these samples exhibited surface carbonate peaks of similar relative intensities (Supplementary Fig. S4b ). Thus, the absence of surface carbonate peaks for LaPrO 3+x @5Li 2 CO 3 under in-situ Raman is more likely due to temperature effect rather than the Li 2 CO 3 loading effect. Fig. 2: In-situ Raman for LaPrO 3+x and LaPrO 3+x @5Li 2 CO 3 . In-situ Raman for a LaPrO 3+x reduction at 700 °C, b LaPrO 3+x reoxidation at 700 °C, c LaPrO 3+x @5Li 2 CO 3 reduction at 700 °C, d LaPrO 3+x @5Li 2 CO 3 reoxidation at 700 °C. Full size image Our previous study on chemical looping ethane conversion indicated that the formation of peroxide species from mixed oxides can be linked to the presence of highly reducible cation components [38] . Therefore, the oxidation states of the Pr cations in the oxidized LaPrO 3+x and LaPrO 3+x @5Li 2 CO 3 mixed oxide catalysts were determined by ex-situ XANES first. It was shown that both Pr 3+ and Pr 4+ are present for the LaPrO 3+x and LaPrO 3+x @5Li 2 CO 3 catalysts (Supplementary Fig. S5 ) [42] . It is evident that LaPrO 3+x @5Li 2 CO 3 contains more bulk Pr 4+ than LaPrO 3+x . The corresponding in-situ XPS measurement also detected the presence of near-surface Pr 4+ and peroxide species. 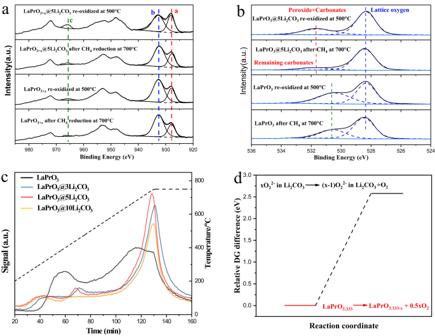Fig. 3: Probe of oxygen species evolution. In-situ XPS spectra on LaPrO3+xand LaPrO3+x@5Li2CO3after methane reduction and oxidation treatments: methane reduction was conducted at 700 °C and re-oxidation was conducted at 500 °C:aandbshow Pr 4fand O 1speaks, respectively;cO2-TPD from LaPrO3+xand LaPrO3+x@Li2CO3with different Li2CO3loadings;dRelative ∆G difference of O2release from LaPrO3.33and Li2O2in amorphous Li2CO3. Figure 3a shows the Pr 3d XPS spectra of LaPrO 3+x and LaPrO 3+x @5Li 2 CO 3 . Although the quantification of Pr 4+ /Pr 3+ with XPS is complex, Sinev et al. have reported the characteristic peaks and features for Pr 4+ with in-situ XPS by switching between oxidizing and reducing atmospheres on a Pr-Ce mixed oxide [43] . A large “a/b” peak area ratio and a large “c” peak area are representative of the Pr 4+ features (as labeled in Fig. 3a ). As shown in Fig. 3a , LaPrO 3+x @5Li 2 CO 3 exhibited much more intense Pr 4+ features than LaPrO 3+x in its oxidized state, confirming the abundance of Pr 4+ in the near surface region in the presence of the Li 2 CO 3 coating. It is noteworthy that Pr 4+ in the near surface region of LaPrO 3+x @5Li 2 CO 3 is largely transformed into Pr 3+ after contacting methane, as indicated by the decreased “c” peak area and “a/b” peak area ratio. In comparison, the changes in the Pr 4+ features were quite unremarkable in Li-free LaPrO 3+x when exposed to methane. This is likely related to spontaneous decomposition of LaPrO 3+x via the reduction of Pr 4+ in the surface region without the Li 2 CO 3 layer, under the low oxygen partial pressure in the in-situ XPS (~1 mbar). The corresponding in-situ XPS O 1 s spectra are presented in Fig. 3b . LaPrO 3+x exhibited an O 1 s peak at B.E. 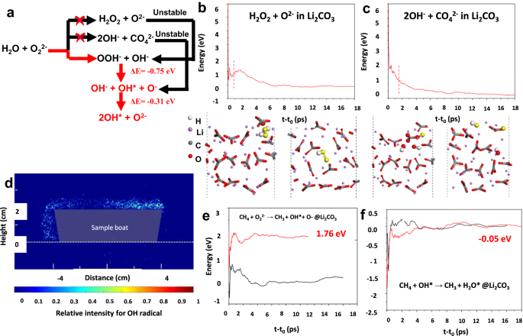Fig. 4: Probe of OH radical evolution. aSummary of the possible reaction product of H2O + O22−;b,c: Mean energies as a function of elapsed time (t-t0) for evolution of H2O2+ O2−and OH−+ CO42−in molten Li2CO3, respectively. The electrophilic oxygen atoms that are involved in the reactions are highlighted in yellow to provide better visualization;dLIF experiments on SiO2@5Li2CO3, scale bar shows the relative intensity for OH radical;eandf:, respectively. = at 528.2 eV that is assigned to lattice oxygen species. The shoulder O 1 s peak at B.E. = 530.7 eV for LaPrO 3+x has not been reported previously. It is thought to arise from stable hydroxyls to the bare LaPrO 3+x since it is independent of the reduction and oxidation treatments. LaPrO 3+x @5Li 2 CO 3 showed two XPS O 1 s peaks: B.E. = 528.2 eV, which corresponds to lattice oxygen and does not vary substantially upon reduction or oxidation; and B.E. = 531.8 eV, which is consistent with previous literature assignments of peroxide [37] . This assignment for peroxide is further substantiated by the fact that it decreased substantially when contacting methane, and increased upon re-oxidation with O 2 . In-situ FTIR-DRIFTS on LaPrO 3+x @5Li 2 CO 3 further confirmed that the carbonate peak increased when methane was injected onto the sample (Supplementary Fig. S6 ). The abundance of peroxide species in LaPrO 3+x @5Li 2 CO 3 , and their absence in LaPrO 3+x , can be explained by: (a) the presence of the Li 2 CO 3 /Li 2 O layer, which inhibits peroxide decomposition into molecular O 2 from the surface of LaPrO 3+x and (b) the increased presence of Pr 4+ compared to LaPrO 3+x as confirmed by XANES and in-situ XPS, which favors O 2 2- formation. Fig. 3: Probe of oxygen species evolution. In-situ XPS spectra on LaPrO 3+x and LaPrO 3+x @5Li 2 CO 3 after methane reduction and oxidation treatments: methane reduction was conducted at 700 °C and re-oxidation was conducted at 500 °C: a and b show Pr 4 f and O 1 s peaks, respectively; c O 2 -TPD from LaPrO 3+x and LaPrO 3+x @Li 2 CO 3 with different Li 2 CO 3 loadings; d Relative ∆G difference of O 2 release from LaPrO 3.33 and Li 2 O 2 in amorphous Li 2 CO 3 . Full size image The stoichiometric x value in Li-free LaPrO 3+x was determined to be 0.33 by thermogravimetric analysis (TGA) upon methane reduction at 700 °C (Supplementary Fig. S7 ). O 2 -TPD were further conducted on LaPrO 3+x and LaPrO 3+x @5Li 2 CO 3 (Fig. 3c ), showing that LaPrO 3+x exhibited substantial O 2 release at much lower temperatures than LaPrO 3+x @5Li 2 CO 3 . Meanwhile, LaPrO 3+x @Li 2 CO 3 with 3–10 wt.% Li 2 CO 3 loadings all exhibited a primary O 2 release peak at ~750 °C. The suppressed peroxide decomposition to gaseous molecular O 2 was further examined via ab-initio molecular dynamics (AIMD). As shown in Fig. 3d , O 2 formation from LaPrO 3+x without the Li 2 CO 3 shell is far more facile than gaseous molecular O 2 formation from Li 2 O 2 in the amorphous Li 2 CO 3 thin film. The detailed structural changes of both reactions are shown in Supplementary Fig. S8 . This is consistent with the higher oxygen release peak temperature in Fig. 3c and indicates that the Li 2 CO 3 layer stabilizes the O 2 2− peroxide species formed from LaPrO 3+x . Furthermore, Li 2 CO 3 has been shown to have a substantial solubility of O 2 2− peroxide species [38] . Active redox species and reaction pathway A detailed AIMD study was conducted to determine the fate of peroxide in Li 2 CO 3 . Interaction between O 2 2− and water has been reported to yield OH radicals (OH * ) in OCM reactions [37] . We further investigated groups of possible products and corresponding reaction pathways using AIMD. As can be seen in Fig. 4a , peroxide is more favorable to evolve into hydroxyl radicals by interacting with H 2 O dissolved in the salt. Clearly, H 2 O 2 + O 2− and 2OH − + CO 4 2− cannot be stable because they spontaneously convert to OOH − + OH − (Fig. 4b ) and OH − + OH * + O − (Fig. 4c ), respectively. It was calculated that OH − + OH * + O − can further evolve into 2OH * + O 2− , intensifying OH * production. This was confirmed with LIF experiments on Li 2 CO 3 coated SiO 2 as a model material at 700°C under O 2 and steam, which can detect the formation of OH * (Fig. 4d ). The interactions between active species and methane were further studied. It was demonstrated that direct C-H bond activation in methane by O 2 2− is not energetically favorable (Fig. 4e ). In comparison, the as-formed hydroxyl radical is highly active for methane activation (Fig. 4f ). This is also consistent with previous literature report on Mn-Na 2 WO 4 /SiO 2 catalysts [44] . Based on the abovementioned experimental and simulation results, the reaction pathway involves peroxide formation on the LaPrO 3+x surface resulting from Pr 4+ → Pr 3+ transition, dissolution of the O 2 2− in the carbonate phase, and subsequent hydroxyl radical formation and CH 3 radical formation by C-H bond cleavage. The surface initiated radical reaction will further drive C 2+ formation in the gas phase [45] . Fig. 4: Probe of OH radical evolution. a Summary of the possible reaction product of H 2 O + O 2 2− ; b , c : Mean energies as a function of elapsed time ( t-t 0 ) for evolution of H 2 O 2 + O 2− and OH − + CO 4 2− in molten Li 2 CO 3 , respectively. The electrophilic oxygen atoms that are involved in the reactions are highlighted in yellow to provide better visualization; d LIF experiments on SiO 2 @5Li 2 CO 3 , scale bar shows the relative intensity for OH radical; e and f :, respectively. Full size image Catalyst reactivity performance for OCM The Li-free LaPrO 3+x exhibited 57.6% methane conversion, but only 5.14% C 2+ selectivity with CO 2 as the main product at 700°C and 1050 hr −1 gas hourly space velocity (GHSV). Li 2 CO 3 promotion significantly increases the C 2+ selectivity of LaPrO 3+x . 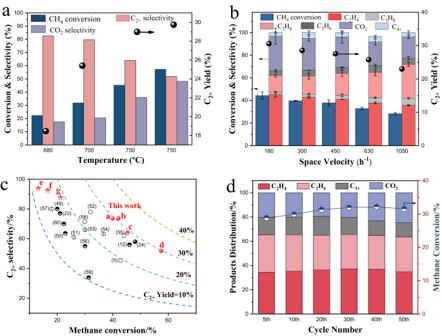Fig. 5: Li2CO3coated LaPrO3+xas a redox catalyst for CL-OCM. Catalyst performance for CL-OCM:aTemperature effect for LaPrO3+x@5Li2CO3:PCH4= 0.4,GHSV= 1050 h−1;bSpace velocity effect for LaPrO3+x@5Li2CO3:T= 700 °C,PCH4= 1.0; The error bars were expressed as the standard deviations of triplicate experiments.cComparison of LaPrO3+x@5Li2CO3with previously reported OCM catalysts: full-filled, half-filled and empty dots representPCH4= 0.8–1, 0.4–0.8 and <0.4 atm, respectively. Seven data points from this work are included:aT= 700 °C,PCH4= 1.0 atm,GHSV= 180 h−1;bT= 700 °C,PCH4= 1.0 atm,GHSV= 300 h−1;cT= 730°C,PCH4= 0.4 atm,GHSV= 1050 h−1;dT= 750°C,PCH4= 1.0 atm,GHSV= 180 h−1;e–gstands for a Mn-Na2WO4/SiO2catalyst tested under a redox mode atPCH4= 0.4 atm andGHSV= 1050 h−1, with reaction temperature = 700, 750 and 800° respectively;d50-redox cycle test on LaPrO3+x@5Li2CO3:T= 700 °C,PCH4= 0.4,GHSV= 1050 h−1. 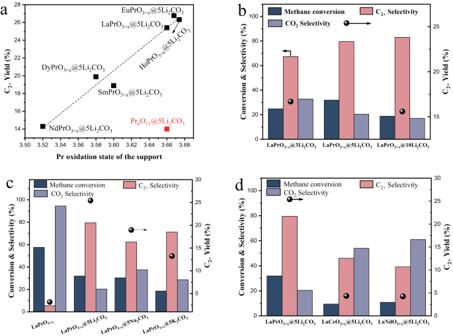Fig. 6: Extension of the LaPrO3+x@5Li2CO3redox catalyst. aPlots of C2+yields with Pr oxidation states of different mixed lanthanide oxide supports;bRedox OCM performance comparison of LaPrO3+x@3Li2CO3, LaPrO3+x@5Li2CO3and LaPrO3+x@10Li2CO3;cRedox OCM performance comparison of LaPrO3+x, LaPrO3+x@Li2CO3, LaPrO3+x@5Na2CO3and LaPrO3+x@5K2CO3;dRedox OCM performance comparison of LaPrO3+x@5Li2CO3, LaCeO3+x@5Li2CO3and LaNdO3+x@5Li2CO3. Reaction conditions forb–d:T= 700 °C,PCH4= 0.4 atm,GHSV= 1050 h−1. Figure 5 summarizes the effects of reaction temperature, space velocity, and methane partial pressure for LaPrO 3+x @5Li 2 CO 3 . Higher temperature led to higher methane conversion and C 2+ yield, but with increased CO 2 selectivity (Fig. 5a ). At 700 °C under pure methane (P CH4 = 1 atm), decreasing GHSV led to increased methane conversions, with only a slight decrease in C 2+ selectivity (Fig. 5b ). A maximum C 2+ yield of 30.6% was obtained at 180 h −1 , the lowest GHSV tested due to instrumentation limitations. The effect of the OCM step duration was investigated, with the optimum duration determined to be 60 s under the current reactor setting. Longer OCM steps decreased methane conversion, while shorter steps reduced C 2+ selectivity (Supplementary Fig. S9 ). We note that the results at all GHSV investigated exceeded the generally accepted “100% rule” for OCM, namely that the sum of methane conversion and C 2+ selectivity does not exceed 100% [46] . The ability to use undiluted methane represents another advantage from a practical standpoint, when compared to most of the previous literature studies that employed significant amounts of diluent. The effect of methane partial pressure was further illustrated in Supplementary Fig. S10 . As can be seen, the space-time yield for ethane, ethylene and CO 2 increased almost linearly with increased methane partial pressure from 0.2 atm to 1.5 atm. This suggests a first-order kinetics for both C 2 and CO x formation. Therefore, the LaPrO 3+x @5Li 2 CO 3 redox catalyst can operate at elevated methane partial pressures, which would be highly beneficial for downstream separation and processing of the C 2+ products. We also note that many of the previously reported OCM catalysts suffered from severe yield penalty at elevated methane partial pressures [26] , [47] , [48] . These findings highlight the advantages of LaPrO 3+x @5Li 2 CO 3 in CL-OCM. Figure 5c compares LaPrO 3+x @5Li 2 CO 3 with previously reported OCM catalysts [49] , [50] , [51] , [52] , [53] , [54] , [55] , [56] , [57] , [58] , [59] , [60] : LaPrO 3+x @5Li 2 CO 3 exhibited the highest OCM yield reported so far, and is the only catalyst that exceeds the 30% single-pass C 2+ yield at 100% methane partial pressure. The optimal operating temperature at 700 °C is also significantly lower than the classical OCM catalysts such as Mn-Na 2 WO 4 /SiO 2 , which exhibits optimal performance at ~850 °C. Traditional Mn-Na 2 WO 4 /SiO 2 catalyst was also synthesized and tested under redox OCM to compare with LaPrO 3+x @5Li 2 CO 3 . C 2+ yields of 12.4%, 15.4% and 18.6% were observed at 700, 750 and 800 °C respectively, indicating that LaPrO 3+x @5Li 2 CO 3 is superior especially at lower reaction temperatures. The LaPrO 3+x @5Li 2 CO 3 catalyst exhibited excellent catalyst stability, as confirmed by long-term performance tests at 700 °C and 1050 h −1 GHSV. Both methane conversion and C 2+ selectivity were stable within 50 redox cycles as shown in Fig. 5d . In comparison, Li/MgO tends to deactivate after contacting methane and O 2 at 750 °C [34] . The high stability of LaPrO 3+x @5Li 2 CO 3 is ascribed to the preservation of the amorphous Li 2 CO 3 overlayer. This was confirmed via ex-situ XPS. As can be seen in Supplementary Fig. S11 , the carbonate O 1 s peak portion for LaPrO 3+x @5Li 2 CO 3 does not decrease after redox cycles, indicating that surface Li 2 CO 3 is maintained. This was also separately validated via a TGA based cyclic experiment (Supplementary Fig. S12 ). This is substantially different from literature reports on Li/MgO, where Li content decreased from 3.1 wt.% to ~0.1 wt.% within 20 h [61] . The preservation of Li in LaPrO 3+x @5Li 2 CO 3 is likely due to the lower reaction temperature and the abundance of Li 2 CO 3 relative to LiOH, thereby inhibiting Li evaporation [10] . Carbon deposition was negligible after the long-term cycle, as proven by the absence of CO and CO 2 during the re-oxidation step (Supplementary Fig. S13 ). We also note that under the reaction temperature, Li 2 CO 3 could partially decompose into Li 2 O, while the as-formed Li 2 O can react with the by-product CO 2 in the OCM step and re-form Li 2 CO 3 . Thus, the catalyst surface is likely to be in a mixed state of Li 2 CO 3 and Li 2 O at any reaction stage. This is proven by using LiNO 3 instead of Li 2 CO 3 for wet impregnation onto LaPrO 3+x , while keeping the same Li amount. The as-synthesized LaPrO 3+x @Li 2 O (after nitrate decomposition) started to exhibit activity for OCM after a few reaction cycles, although the C 2+ yield is lower than that of LaPrO 3+x @Li 2 CO 3 (Supplementary Fig. S14 ). The presence of Li 2 O in Li 2 CO 3 can be beneficial for the formation of Li 2 O 2 by reacting with the active oxygen species on the LaPrO 3+x surface. Fig. 5: Li 2 CO 3 coated LaPrO 3+x as a redox catalyst for CL-OCM. Catalyst performance for CL-OCM: a Temperature effect for LaPrO 3+x @5Li 2 CO 3 : P CH4 = 0.4, GHSV = 1050 h −1 ; b Space velocity effect for LaPrO 3+x @5Li 2 CO 3 : T = 700 °C, P CH4 = 1.0; The error bars were expressed as the standard deviations of triplicate experiments. c Comparison of LaPrO 3+x @5Li 2 CO 3 with previously reported OCM catalysts: full-filled, half-filled and empty dots represent P CH4 = 0.8–1, 0.4–0.8 and <0.4 atm, respectively. Seven data points from this work are included: a T = 700 °C, P CH4 = 1.0 atm, GHSV = 180 h −1 ; b T = 700 °C, P CH4 = 1.0 atm, GHSV = 300 h −1 ; c T = 730°C, P CH4 = 0.4 atm, GHSV = 1050 h −1 ; d T = 750°C, P CH4 = 1.0 atm, GHSV = 180 h −1 ; e – g stands for a Mn-Na 2 WO 4 /SiO 2 catalyst tested under a redox mode at P CH4 = 0.4 atm and GHSV = 1050 h −1 , with reaction temperature = 700, 750 and 800° respectively; d 50-redox cycle test on LaPrO 3+x @5Li 2 CO 3 : T = 700 °C, P CH4 = 0.4, GHSV = 1050 h −1 . Full size image Generalizability of the OCM catalyst design strategy The core-shell redox catalyst design strategy can be extended to other Pr-containing mixed lanthanide oxides. NdPrO 3+x , DyPrO 3+x , SmPrO 3+x , HoPrO 3+x and EuPrO 3+x were synthesized using a similar method. The Pr oxidation states of the carbonate-free mixed oxides were determined by TGA measurement of oxygen stoichiometry upon methane reduction at 700 °C. The mixed oxides were then loaded with 5 wt.% Li 2 CO 3 and examined for OCM. The C 2+ yields, plotted in Fig. 6a , correspond to the Pr oxidation state in the mixed oxides. A linear relationship is observed between the C 2+ yield and the initial Pr oxidation state. EuPrO 3+x @5Li 2 CO 3 and HoPrO 3+x @5Li 2 CO 3 even achieved slightly better C 2+ yields than LaPrO 3+x @5Li 2 CO 3 . The significantly reduced C 2+ yield of Pr 6 O 11 @5Li 2 CO 3 , despite the Pr oxidation state in Pr 6 O 11 being +3.67, can be attributed to the instability of the Pr 6 O 11 phase in the presence of Li 2 CO 3 . This leads to the formation of the Li 26 Pr 36 O 73 phase after cycling. (see Supplementary Fig. S15a ) and consistent with the report by Aono et al., who observed the same phase by heating up the a Pr 6 O 11 and Li 2 CO 3 mixture [62] . The decrease in the Pr oxidation state and disruption of the Li 2 CO 3 layer renders low C 2+ yield. In comparison, all the Li 2 CO 3 promoted mixed lanthanide oxides, which the exception of NdPrO 3+x , maintained their original phases after cycling, and no Li-containing phases were observed (Supplementary Figs. S15 b–e). This also highlights the importance of the secondary rare earth metal cation such as La and Sm, which stabilizes Pr 4+ and inhibits the solid-state reaction with the Li 2 CO 3 promoter. The Li 2 CO 3 loading effect on LaPrO 3+x was also investigated as shown in Fig. 6b . Although the oxygen release behaviors were all substantially altered with different Li 2 CO 3 loadings as shown in O 2 -TPD (Fig. 3c ), the loading amount exhibits an optimum and LaPrO 3+x @5Li 2 CO 3 achieved the highest C 2+ yield. In addition to Li 2 CO 3 , other alkali metal carbonate promoters including Na 2 CO 3 and K 2 CO 3 were also investigated as shown in Fig. 6c . Switching from Li 2 CO 3 to Na 2 CO 3 and K 2 CO 3 leads to decreased catalyst activities and decreased C 2+ yields. This may be due to the lower activities of Na 2 O 2 and K 2 O 2 , where Na 2 O 2 and K 2 O 2 are more thermodynamically stable than Li 2 O 2 (Supplementary Table S2 ). The necessity of Pr in the mixed metal oxide support was also investigated by switching Pr to Ce and Nd, where Ce and Nd locating very close to Pr in the periodic table in the lanthanide family. As shown in Fig. 6d , both LaCeO 3+x @5Li 2 CO 3 and LaNdO 3+x @5Li 2 CO 3 exhibited very low C 2+ yields and high selectivities towards CO 2 . This is probably due to the properties of the Pr 4+ ↔Pr 3+ redox pair, which leads to efficient generation of peroxide oxygen species in the Li 2 CO 3 salt. Fig. 6: Extension of the LaPrO 3+x @5Li 2 CO 3 redox catalyst. a Plots of C 2+ yields with Pr oxidation states of different mixed lanthanide oxide supports; b Redox OCM performance comparison of LaPrO 3+x @3Li 2 CO 3 , LaPrO 3+x @5Li 2 CO 3 and LaPrO 3+x @10Li 2 CO 3 ; c Redox OCM performance comparison of LaPrO 3+x , LaPrO 3+x @Li 2 CO 3 , LaPrO 3+x @5Na 2 CO 3 and LaPrO 3+x @5K 2 CO 3 ; d Redox OCM performance comparison of LaPrO 3+x @5Li 2 CO 3 , LaCeO 3+x @5Li 2 CO 3 and LaNdO 3+x @5Li 2 CO 3 . Reaction conditions for b – d : T = 700 °C, P CH4 = 0.4 atm, GHSV = 1050 h −1 . Full size image In this work, we present a generalized strategy for the chemical looping - oxidative coupling of methane (CL-OCM) using Li 2 CO 3 -promoted mixed rare earth oxides. A detailed study on LaPrO 3+x @Li 2 CO 3 revealed a single-pass C 2+ yield of up to 30.6% with good catalyst stability at 700°C. Additionally, the operational partial pressure of methane can exceed 1 atm, offering potential industrial benefits. The Li 2 CO 3 promotion formed a surface layer on LaPrO 3+x , increasing both the bulk and surface Pr 4+ contents, which in turn enhanced OCM activity. This finding was corroborated by ex-situ XANES, in-situ Raman, in-situ XRD, and in-situ XPS analyses. In-situ Raman and XPS measurements also suggested that Pr 4+ contributed to the presence of near surface peroxide on LaPrO 3+x @Li 2 CO 3 . The peroxide species would subsequently transform into hydroxyl radicals for methane activation, as supported by both LIF experiments and AIMD simulations. A generalized correlation between the oxidation state of Pr in the mixed lanthanide oxide and C 2+ yield was also observed, providing a valuable strategy for optimizing this family of OCM catalysts. Given their high yields and favorable operational parameters, Li 2 CO 3 -promoted mixed rare earth oxides hold great promise for the direct conversion of methane to C 2+ products. Redox catalyst preparation A modified Pechini method was used to prepare LaPrO 3+x . Stoichiometric amounts of La(NO 3 ) 9 ·6H 2 O (99.0%, Sigma-Aldrich, 10 g) and Pr(NO 3 ) 9 ·6H 2 O (99.0%, Sigma-Aldrich, 10 g) were dissolved in 100 ml deionized water and stirred to form a transparent solution. Citric acid (99.5%, Sigma-Aldrich, 28 g) at a 3:1 molar ratio to metal ions, and ethylene glycol (99.8%, Sigma-Aldrich, 18 ml) at a 2:1 molar ratio to citric acid were added into the solution. The obtained solution was stirred constantly at 80 °C to form a viscous gel. After that, the gel was transferred to a convection oven for drying at 130 °C overnight and was then calcined in a tube furnace at 850 °C for 8 h. A wet impregnation method was used to synthesize LaPrO 3+x @Li 2 CO 3 . Calculated amount of Li 2 CO 3 (ACS reagent; ≥99.0%) was dissolved in 10 ml deionized water. 5 g of LaPrO 3+x was added into the solution under stirring. After drying at 130 °C for 2 h, the dried particles were calcined in a furnace at 750 °C for 3 h. Finally, the powders were ground, pressed and crushed into 60–80 mesh as final LaPrO 3+x @Li 2 CO 3 . Redox catalyst characterization Redox catalyst surface and morphology characterizations were conducted with ex-situ and in-situ XRD, ex-situ and in-situ XPS, ex-situ and in-situ S/TEM, in-situ Raman, quasi in-situ LEIS, in-situ DRIFTS-FTIR and ex-situ XANES. Ex-situ XRD was conducted with a Rigaku SmartLab X-ray diffractometer at NC State University. In-situ XRD was conducted on an Empyrean X-ray diffractometer equipped with an Anton-Paar XRK-900 reactor chamber at NC State University. Ex-situ XPS was conducted on an ESCALAB 250Xi (Thermo Fisher) at Guangzhou Institute of Energy Conversion. In-situ XPS was conducted with SPECS EnviroESCA at Dalian Institute of Chemical Physics. S/TEM were conducted on an aberration corrected Thermo Scientific Titan 80-300 STEM at NC State University. In-situ Raman was conducted on a Horiba LabRam-HR Raman spectrometer at Lehigh University. Quasi in-situ HS-LEIS was conducted at the Surface Analysis Center at Lehigh University with an ION-TOF Qtac 100 for outermost surface layer compositional analysis and depth profiling. In-situ DRIFTS-FTIR was conducted on a Thermo Fisher Nicolet iS50 FTIR equipped with a DiffusIR sample chamber (Pike Technologies) at NC State University. Ex-situ XANES was conducted on an X-ray Absorption Fine structure for catalysis (XAFCA) with an ion-chamber detector at Singapore Synchrotron Light Source. Characterization details of each method can be found in the supplemental document. Reactivity tests Reactivity tests were conducted in a fixed bed quartz U-tube reactor with ID of 1/8 inches or 3.18 mm. Approximately 2 g of catalyst was loaded at the bottom of the U-tube reactor with quartz wool placed on both sides of the reactor to keep the catalysts in place. Typically, the OCM reaction was conducted at 700 °C, a mixture of methane (20–100%, balance Ar) was injected into the reactor for 1 min. After the OCM step, Ar was introduced to purge the reactor for 5 min and then 10% oxygen (5 mL/min, balance Ar) was introduced for the oxidation step for 3 min. A gas bag was used to collect all the gas product over the entire OCM step. The obtained gaseous products collected were detected by gas chromatography (Agilent 7890 A). To confirm the redox stability of the redox catalyst, 50 reduction and oxidation steps were performed following the above procedure, with 5 min of Ar purge in between. The catalyst OCM activity are calculated based on the average products across the OCM step obtained in the gas bag. The equations used for calculating conversions, selectivities and yields are: 
    Methane Conversion= Methane Input -Methane Output/Methane Input
 (1) 
    C2+ Selectivity=moles of C in C2+ products/moles of C in converted methane
 (2) 
    C2+ Yield=Methane Conversion ∗ Selectivity of C2+
 (3) Computational details AIMD calculations were implemented by the Vienna ab initio Simulation package (VASP) with the frozen-core all-electron projector augmented wave (PAW) model and Perdew-Burke-Ernzerhof (PBE) functions. A kinetic energy cutoff of 350 eV is used for the plane-wave expansion of the electronic wave function, and a Γ-point is chosen for sampling the first Brillouin zone. The convergence criteria of force and energy were set to 0.01 eV/Å and 10 −5 eV respectively. The strong on-site coulomb interaction on the d-orbital electrons on the Fe sites is treated with the generalized gradient approximation (GGA) + U approach with U eff = 4 eV for the f-orbital of Pr. Spin polarization is included in all calculations. Constant temperature AIMD simulations are performed at 1000 K, which is slightly above the experimental reaction temperature (700 °C). The atomic motions are treated classically and propagated with 1 fs time steps. The internal energy of all molten systems is obtained from the AIMD simulations as the time average kinetic and potential energy: \(E\left(t\right)=\frac{1}{t-{t}_{0}}{\int }_{{t}_{0}}^{t}\left({E}_{{DFT}}\left(\tau \right)+{E}_{{kin}}\left(\tau \right)\right)d\tau\) [6] , where \({t}_{0}\) is chosen to allow the system to equilibrate and lose memory of the initial conditions, which was set as 10 ps unless otherwise stated. For the gas-molecules, \(E\left(t\right)\) are corrected by adding the translational energy \(\frac{3}{2}{k}_{B}T\) because it contains only rotational and vibrational contributions, where k B is the Boltzmann constant. The estimated change in Gibbs free energy is obtained as \(\varDelta {G}_{{estimate}}^{^\circ }=\varDelta E+p\varDelta V-T\varDelta {S}_{{estimate}}^{^\circ }\) , where the volume change ( \(\varDelta V\) ) is assumed to originate purely from changes in the number of gas phase molecules ( \(\varDelta {n}_{{gas}}\) ) and is calculated by the ideal gas law ( \(p\varDelta V=\varDelta {n}_{{gas}}{k}_{B}T\) ). The entropies of the studied radicals are obtained from NIST.